Fat, fibre and cancer risk in African Americans and rural Africans Rates of colon cancer are much higher in African Americans (65:100,000) than in rural South Africans (<5:100,000). The higher rates are associated with higher animal protein and fat, and lower fibre consumption, higher colonic secondary bile acids, lower colonic short-chain fatty acid quantities and higher mucosal proliferative biomarkers of cancer risk in otherwise healthy middle-aged volunteers. Here we investigate further the role of fat and fibre in this association. We performed 2-week food exchanges in subjects from the same populations, where African Americans were fed a high-fibre, low-fat African-style diet and rural Africans a high-fat, low-fibre western-style diet, under close supervision. In comparison with their usual diets, the food changes resulted in remarkable reciprocal changes in mucosal biomarkers of cancer risk and in aspects of the microbiota and metabolome known to affect cancer risk, best illustrated by increased saccharolytic fermentation and butyrogenesis, and suppressed secondary bile acid synthesis in the African Americans. In the west, colon cancer is the second leading cause of cancer death. It afflicts ∼ 150,000 Americans, 250,000 Europeans and 1 million people worldwide annually. Nearly one third will die [1] . Colonoscopy has permitted early detection and recent studies have shown this to be associated with a reduction in mortality rates, but overall impact has been small, particularly among African Americans who shoulder the greatest burden of the disease in the United States. Colon cancer is one of the westernized diseases, with an incidence in Americans of African descent of 65:100,000 compared with <5:100,000 in rural Africans. Migrant studies, such as those in Japanese Hawaiians, have demonstrated that it only takes one generation for the immigrant population to assume the colon cancer incidence of the host western population [2] . Although the change in diet is most probably responsible for this [3] , migration changes many other aspects of the environment. For example, cigarettes, chemicals, infections and antibiotics might be equally responsible for the change in colon cancer risk. To focus on the importance of diet in African Americans and to explore the hypothesis that colon cancer risk is determined by the influence of the diet on the microbiota to produce anti- or pro-neoplastic metabolites, we have performed a series of investigations between African Americans and rural South Africans [4] , [5] . First, we observed that their diets were fundamentally different in preparation, cooking and composition. Animal protein and fat intake was two to three times higher in Americans, whereas carbohydrate and fibre, chiefly in the form of resistant starch, were higher in Africans. On colonoscopy, African Americans had more polyps and higher rates of mucosal proliferation, measured by Ki67 epithelial cell staining, confirming its potential use as a biomarker of cancer risk [6] . These differences were shown to be associated with profound differences in the microbiota (Americans dominated by genus Bacteroides and Africans by the genus Prevotella ) and metabolic phenotype. Notable differences included higher levels of starch degraders, carbohydrate fermenters and butyrate producers and their metabolites in Africans, and higher levels of potentially pathogenic proteobacteria ( Escherichia and Acinetobacter ) and bile acid deconjugators and their products in Americans [5] . As there is extensive experimental evidence that the products of fibre fermentation, in particular butyrate, are anti-inflammatory and anti-neoplastic [7] , [8] , [9] , and that the products of bacterial bile acid conjugation, secondary bile acids, are carcinogenic [10] , these findings suggested two potential mechanisms for diet-associated cancer risk: the protective effect of dietary fibre in increasing butyrogenesis and the promotional effect of dietary fat on stimulating bile acid synthesis by the liver. We know from the results of two recently published human studies that modifications of the fibre and fat content of the diets have a major impact on the colonic microbiota within a few days [11] , [12] . Here we provide critical information on the functional significance of these microbiota changes on the colonic mucosa by switching the fat and fibre proportions of the diet in our two high and low colon cancer risk study populations. 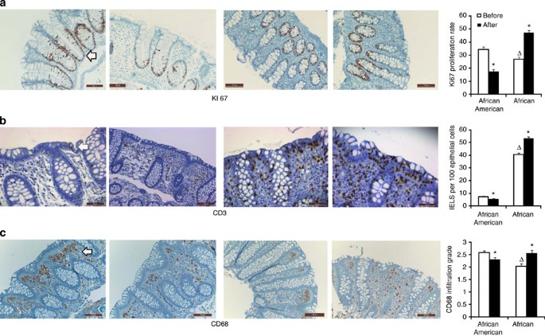Figure 1: Colonic mucosal immunohistochemistry of proliferative and inflammatory biomarkers. Immunohistochemical analysis of colonic mucosal biopsies taken at colonoscopy with their associated quantitative analysis on the right panel. (a) An illustration of the paired changes in Ki67 staining of epithelial crypt cells in one African American (the first and second panels) and one rural African (the third and 4th panels left to right) before and after dietary switch. (b) Paired changes in CD3+staining, similar toa. (c) Paired changes in CD68+macrophages in the lamina propria. The bar graphs on the far right summarize the group mean±s.e. results in 20 African Americans and 12 rural Africans. The two-tailed Mann–WhitneyU-test was used for comparisons for non-paired samples and the Wilcoxon rank sum test for paired samples, with Bonferroni correction for multivariate comparisons. Triangles indicate significant (P<0.05) baseline differences and stars indicate significant changes induced by diet switch. Employing the study design outlined on Table 1 , we showed the anticipated increase in saccharolytic fermentation and butyrogenesis, and suppression of secondary bile acid synthesis produced by switching African Americans to a high-fibre, low-fat diet for 2 weeks, were associated with a significant reduction in colonic mucosal inflammation and proliferation biomarkers of cancer risk. In stark contrast, the diet switch in rural Africans to a high-fat, low-fibre diet resulted in reverse changes in all these parameters. Table 1 Study design, time schedule and sampling. Full size table Changes in the colonic mucosa following diet switch Measurements made in the home environment (HE) confirmed our preceding studies that the dietary intakes were quite different, with animal protein and fat intake being two to three times higher in Americans and fibre intake, chiefly in the form of resistant starch, being higher in Africans [4] ( Supplementary Fig. 1 and Supplementary Tables 1–3 ). On colonoscopy, adenomatous polyps were found and removed in nine Americans and no Africans. Measurements of mucosal epithelial proliferation rates by Ki67 staining of biopsies from ascending, transverse and descending colon, all showed significantly higher levels in African Americans than in Africans ( Fig. 1 and Supplementary Fig. 2 ), again supporting its use as a biomarker of cancer risk. The dietary switch was well tolerated by both populations and body weights were all maintained with 2 kg. Remarkably, the switch decreased proliferative rates in African Americans to levels lower than those of Africans at baseline, whereas rates increased in Africans to levels greater than African Americans at baseline ( Fig. 1 ). In tandem, histological ( Supplementary Tables 5a–d ) and immunohistochemical markers of inflammation ( Fig. 1b,c ) used, namely CD3 + intraepithelial lymphocytes and CD68+ lamina propria macrophages, increased on switching Africans to the high-fat diet and decreased in Americans given the high-fibre diet, thus parallelling the measured changes in mucosal proliferation. Figure 1: Colonic mucosal immunohistochemistry of proliferative and inflammatory biomarkers. Immunohistochemical analysis of colonic mucosal biopsies taken at colonoscopy with their associated quantitative analysis on the right panel. ( a ) An illustration of the paired changes in Ki67 staining of epithelial crypt cells in one African American (the first and second panels) and one rural African (the third and 4th panels left to right) before and after dietary switch. ( b ) Paired changes in CD3 + staining, similar to a . ( c ) Paired changes in CD68 + macrophages in the lamina propria. The bar graphs on the far right summarize the group mean±s.e. results in 20 African Americans and 12 rural Africans. The two-tailed Mann–Whitney U -test was used for comparisons for non-paired samples and the Wilcoxon rank sum test for paired samples, with Bonferroni correction for multivariate comparisons. Triangles indicate significant ( P <0.05) baseline differences and stars indicate significant changes induced by diet switch. Full size image Changes in colonic microbial metabolism following diet switch The reciprocal changes in mucosal proliferation and inflammation between Africans and Americans were associated with reciprocal changes in specific microbes and their metabolites that support our hypothesis that the mechanism whereby diet affects colon cancer risk is mediated by the microbiota. First, there was strong evidence that butyrogenesis was associated with lower mucosal proliferation, both in Africans consuming their usual high-fibre diet and in African Americans switched to a high-fibre African-style diet ( Figs 1 and 2 , and Supplementary Table 6 ). As a wide variety of microbes have the capacity to produce butyrate, we targeted our analysis on the measurement of microbial genes encoding the final enzyme in butyrogenesis, namely butyryl-coenzyme-A-CoA transferase [13] . On their usual diet, Africans had significantly greater abundances of butyrate synthesizing genes, and higher fecal butyrate concentrations ( Fig. 2 ) and colonic evacuate quantities ( Supplementary Table 7 ), whereas switching them to a western, low-fibre diet suppressed each of these parameters. Reciprocally, our measurements of butyrogenesis were lower in Americans consuming their usual low-fibre diet and increased after dietary switch to a high-fibre African-style diet. Impressively, ‘Africanization’ of the diet increased total quantities of butyrate in colonic evacuates 2.5 times, whereas ‘westernization’ reduced quantities by half. 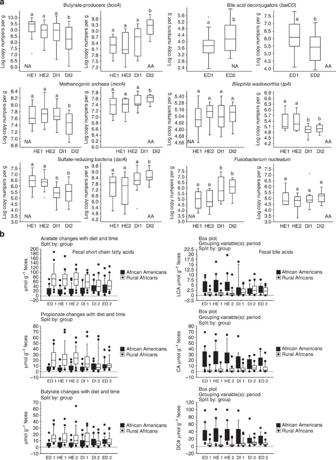Figure 2: Targeted Analysis of microbial functional genes of specific interest and their metabolites. Box plots with whiskers and outliers summarizing the results for the targeted functional quantitative PCR analysis of microbial genes of interest (a) and measurements of their metabolic products in fecal samples (b) in 20 African American (AA) and 20 rural Africans (NA) at sequential time points during the study. Group median and variability outside the upper and lower quartiles are shown. Measurements were taken before (Table 1: ED1, HE1 and HE2), during (DI1 and DI2) and after (ED2) 2 weeks of dietary change. With regard to the functional gene analysis,bcoAcodes for the enzyme butyryl-CoA:acetate CoA-transferase, which is responsible for the last step in butyrate synthesis,mcrAfor the enzyme responsible for methanogenesis,baiCDfor the 7-α-dehydroxylating enzyme responsible for secondary bile acid production, andtpAfor taurine:pyruvate aminotransferase. LCA, lithocholic acid; CA, cholic acid; DCA, deoxycholic acid. As data were not normally distributed, the Kruskal–Wallis test was used to evaluate the significance of the group median differences across the different time points shown on the box plots. In the upper panel, comparison with baseline ED1, ‘a’ signifies no significant change and ‘b’ a significant change. In the lower panel for the short-chain fatty acids acetate, propionate and butyrate, and the secondary bile acids LCA and DCA, and primary bile acid CA, there were no significant differences between time points ED1, HE1 and HE2, while ED2 was consistently different (P<0.05, for details, seeSupplementary Table 6). This, together withSupplementary Fig. 6, illustrates no significant effect from colonoscopy and a profound effect from the dietary change. Figure 2: Targeted Analysis of microbial functional genes of specific interest and their metabolites. Box plots with whiskers and outliers summarizing the results for the targeted functional quantitative PCR analysis of microbial genes of interest ( a ) and measurements of their metabolic products in fecal samples ( b ) in 20 African American (AA) and 20 rural Africans (NA) at sequential time points during the study. Group median and variability outside the upper and lower quartiles are shown. Measurements were taken before ( Table 1 : ED1, HE1 and HE2), during (DI1 and DI2) and after (ED2) 2 weeks of dietary change. With regard to the functional gene analysis, bcoA codes for the enzyme butyryl-CoA:acetate CoA-transferase, which is responsible for the last step in butyrate synthesis, mcrA for the enzyme responsible for methanogenesis, baiCD for the 7-α-dehydroxylating enzyme responsible for secondary bile acid production, and tpA for taurine:pyruvate aminotransferase. LCA, lithocholic acid; CA, cholic acid; DCA, deoxycholic acid. As data were not normally distributed, the Kruskal–Wallis test was used to evaluate the significance of the group median differences across the different time points shown on the box plots. In the upper panel, comparison with baseline ED1, ‘a’ signifies no significant change and ‘b’ a significant change. In the lower panel for the short-chain fatty acids acetate, propionate and butyrate, and the secondary bile acids LCA and DCA, and primary bile acid CA, there were no significant differences between time points ED1, HE1 and HE2, while ED2 was consistently different ( P <0.05, for details, see Supplementary Table 6 ). This, together with Supplementary Fig. 6 , illustrates no significant effect from colonoscopy and a profound effect from the dietary change. Full size image Recognizing that butyrogenesis is a final common pathway of fibre fermentation, which can only be accomplished by multiple microbial metabolic interactions, we examined the simultaneous changes in the group of microbes that remove the major metabolic end product, hydrogen. If hydrogen is allowed to accumulate, it impairs the regeneration of oxidized pyridine nucleotides, which in turn inhibit the fermentation process and butyrogenesis [14] . The efficient removal of hydrogen by the hydrogenotrophic microbes, methanogens, which bind hydrogen into non-toxic methane, sulfate-reducers, which incorporate hydrogen into hydrogen sulfide, and acetogens, which consume hydrogen to produce acetate and water, is therefore a prerequisite for enhanced butyrogenesis. Our observation that all these microbial groups were indeed in greater abundance, as were their metabolic products, both in Africans consuming their usual high-fibre diet and when Americans were switched to the high-fibre diet ( Fig. 2 ) well illustrates the importance of microbial partnership in the maintenance of colonic health. Flint and colleagues [15] have provided strong evidence that the most active butyrate producers, for example, Roseburia spp. and Eubacterium rectale and Faecalibacterium prausnitzii are contained within Clostridium groups IV and XIVa. As Africans and African Americans have very distinct microbiota composition at baseline ( Supplementary Table 8 ), we performed a global analysis of the microbiota by 16S ribosomal RNA gene phylogenetic microarray (Human Intestinal Tract Chip (HITChip)) to examine whether these groups were more prevalent with high fibre consumption [16] . Remarkably, these groups were no more apparent in Africans or Americans eating a high-fibre diet. In fact, the compositional changes that were specifically associated to the diet switch were minor (ten genus-like groups for Africans and two for Americans; Fig. 3a ). These observations suggest either dissociation between structure and function or a change in microbial interactions within the community [17] . On the other hand, we observed stronger co-occurrence patterns between the genus-level taxa in Africans consuming their usual high-fibre diet ( Fig. 3b ), which included these potential butyrate producers, for example, E. rectale et rel. and Clostridium symbiosum et rel., and bacteria associated with complex carbohydrate utilization, for example, Oscillospira guillermondii et rel. Reduction in fibre consumption led to opposite associations ( Fig. 3b , bottom right). Reciprocally, high-fibre feeding in Americans was associated with a shift from correlations between Bacteroides and potential butyrate-producing groups ( Roseburia intestinalis et rel. and C. symbiosum et rel.) towards stronger co-occurrence patterns including Firmicutes that are typically associated with complex carbohydrate fermentation ( Fig. 3b , top right). 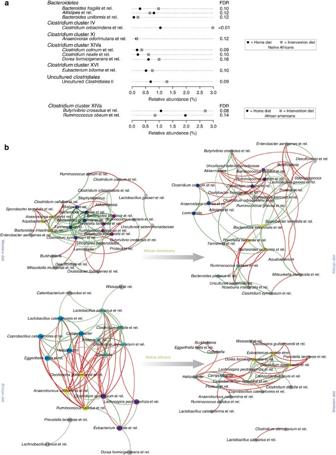Figure 3: The impact of diet switch on microbiota composition and co-occurrence networks. (a) An overview of significantly altered genus-like bacterial groups (FDR<0.2; linear model) following the 14-day diet change. Average fraction of total HITChip signal (proxy for relative abundance) over the samples for each comparison. Black and grey squares indicate the average abundances at home- and intervention diet, respectively. (b) The microbiota genus-like group co-occurrence networks of Africans and African Americans under both dietary regimens for genus-like groups. Groups with correlation differences >1 before and after the diet and at least |r|>0.5 are shown. Positive correlations are indicated with green lines; negative correlations with red lines. Identically coloured nodes indicate network modules with three or more co-occurring groups. Grey nodes represent modules of less than three co-occurring groups or those not represented by a module. The sample sizes are 20 African Americans and 17 rural (Native) Africans. Figure 3: The impact of diet switch on microbiota composition and co-occurrence networks. ( a ) An overview of significantly altered genus-like bacterial groups (FDR<0.2; linear model) following the 14-day diet change. Average fraction of total HITChip signal (proxy for relative abundance) over the samples for each comparison. Black and grey squares indicate the average abundances at home- and intervention diet, respectively. ( b ) The microbiota genus-like group co-occurrence networks of Africans and African Americans under both dietary regimens for genus-like groups. Groups with correlation differences >1 before and after the diet and at least | r |>0.5 are shown. Positive correlations are indicated with green lines; negative correlations with red lines. Identically coloured nodes indicate network modules with three or more co-occurring groups. Grey nodes represent modules of less than three co-occurring groups or those not represented by a module. The sample sizes are 20 African Americans and 17 rural (Native) Africans. Full size image Global changes in the metabonome following diet switch We have described metabonomics and the associated term, metabolomics, as the multiparametric metabolic responses of complex systems to perturbations through time [18] . Specifically, metabonomics addresses such phenotypic changes at the level of small-molecule metabolites and maps these processes using appropriate analytical and statistical processes. Recognizing the extreme complexity of the microbiota and its ability to produce a wide array of other metabolites that could affect mucosal health, we performed compositional and pathway analysis [19] on fecal water and urine samples by 1 H NMR ( Figs 4 and 5 ). Perhaps one of the most striking findings of this study was the dramatically higher quantities and diversity of metabolites in fecal water in Africans consuming their usual diet compared with African Americans ( Fig. 4a ). Although the higher levels of products of saccharolytic fermentation were expected from our targeted analysis, the higher quantities of proteolytic fermentation products were not. The only significantly more abundant fecal metabolite identified in the Americans at baseline, and in Africans after westernization of their diets, was choline. This is highly significant, as recent studies have shown that choline is extensively metabolized by the microbiota to trimethylamine [20] that is absorbed and metabolized by the liver to trimethylamine- N -oxide, which is strongly atherogenic [21] , providing yet another link between westernized diets, the microbiota and westernized diseases. Evidence that this metabolic pathway was indeed stimulated in Africans given the western diet was the observed increase in urine trimethylamine- N -oxide ( Table 2 ). Reciprocal changes in urinary metabolites derived from microbial metabolism of green vegetables, for example,, N -acetyl- S -methyl- L -cysteine sulfoxide, were also observed following diet switch, suggesting that some of the reduction in mucosal proliferation in Americans could also have been related to the effects of increased phytochemical consumption in the Africanized diets [22] . The urinary spectra obtained from African Americans following the change to a high-fibre diet also revealed a marked increase in an unrecoginized metabolite ( Fig. 4a , left upper panel), possibly a nicotinamide breakdown product, whose character and function have yet to be determined. 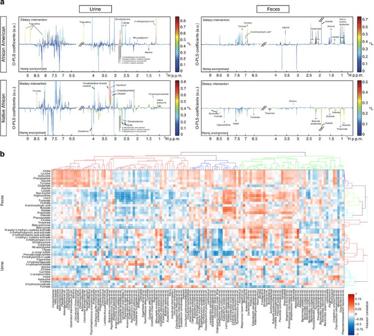Figure 4: The impact of diet switch on fecal and urinary metabolites and their correlation with fecal microbiota. (a)1H NMR fecal and urinary spectra obtained from African Americans (AA) and native Africans (NA) during the home environment period (HE) and post dietary intervention (DI). Metabolites distinguishing the two groups are labelled either above the line (higher after dietary intervention) or below (higher in home environment), and the colour represents the correlation coefficient (r2) of the metabolite with the groups. (b) Two-way clustered heatmap of partial correlation between phylotypes assigned to genus-level taxa whose representation in the fecal microbiota (xaxis) of African American (AA) and rural Africans (NA), and relative metabolite concentrations in urine and feces (yaxis).P-values from correlation were adjusted for multiple testing using the Benjamini–Hochberg FDR. Given a large number of tests performed, a cutoff value of 0.3 was used to define the significance denoted by ‘+’. This level follows the Food and Drug Administration guidelines for bioanalytical biomarkers and was chosen because of the relatively low number of samples it allows for less false negatives. Fecal metabolites (upper compartment) demonstrated a higher number of significant correlations with fecal microbiota compared with urinary metabolites (lower compartment).E. rectale et rel., Lachnospira pectinoschiza et rel., R. intestinalis et rel. and Lactobacillus bovis et rel.correlate strongly with butyrate, acetate and formate. Adjustments were made for country (binary vector with 0=AA and 1=NA) and diet/stage (0=HE 2 and 1=DI 2, see Table 2) in calculating the partial correlations). Figure 4: The impact of diet switch on fecal and urinary metabolites and their correlation with fecal microbiota. ( a ) 1 H NMR fecal and urinary spectra obtained from African Americans (AA) and native Africans (NA) during the home environment period (HE) and post dietary intervention (DI). Metabolites distinguishing the two groups are labelled either above the line (higher after dietary intervention) or below (higher in home environment), and the colour represents the correlation coefficient ( r 2 ) of the metabolite with the groups. ( b ) Two-way clustered heatmap of partial correlation between phylotypes assigned to genus-level taxa whose representation in the fecal microbiota ( x axis) of African American (AA) and rural Africans (NA), and relative metabolite concentrations in urine and feces ( y axis). P -values from correlation were adjusted for multiple testing using the Benjamini–Hochberg FDR. Given a large number of tests performed, a cutoff value of 0.3 was used to define the significance denoted by ‘+’. This level follows the Food and Drug Administration guidelines for bioanalytical biomarkers and was chosen because of the relatively low number of samples it allows for less false negatives. Fecal metabolites (upper compartment) demonstrated a higher number of significant correlations with fecal microbiota compared with urinary metabolites (lower compartment). E. rectale et rel., Lachnospira pectinoschiza et rel., R. intestinalis et rel. and Lactobacillus bovis et rel. correlate strongly with butyrate, acetate and formate. Adjustments were made for country (binary vector with 0=AA and 1=NA) and diet/stage (0=HE 2 and 1=DI 2, see Table 2) in calculating the partial correlations). 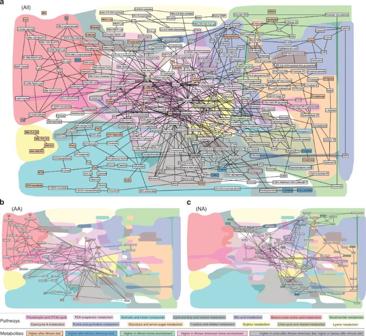Figure 5: The impact of diet switch on fecal and urinary metabolic reaction networks. (a–c) Metabolic reaction networks of metabolites found differentially expressed between different dietary comparisons, created using the MetaboNetworks software19using information from the Kyoto Encyclopaedia of Genes and Genomes (KEGG) on the reactions and enzymes within the biological system. The network shows links between metabolites if the reaction entry in KEGG indicates a main reactant pair and the reaction is either mediated by (1) an enzyme linked to human genes, (2) an enzyme linked to genes from identified bacterial groups using the HITChip or (3) it is part of a spontaneous process. The colour of the metabolites indicate whether the metabolite is found in higher concentrations in the urine/feces of individuals consuming an African diet (orange), higher in individuals consuming an African American diet (blue), higher in the African American home environment (light red), higher in the African home environment (green) or whether the metabolites is not significantly associated with any comparison but is part of the metabolic network (white). Two metabolites (alanine and formate) are found with opposite associations in feces and urine (Table 2), these are therefore represented with a grey background colour. A table with full names for each of the abbreviated metabolite names can be found inSupplementary Table 11. The background shading indicates different interconnected pathways. In the top part of the legend, the colour for each pathway, as represented in the figure, is shown. The bottom part of the legend, with black boxes around text box, indicates the association of each metabolite. (a) Global network of changes (‘All’) observed in fecal water and urine, and in any comparison of the different groups. (b) Network of fecal metabolites found differentially expressed in African Americans before and after the dietary switch (‘AA’). (c) Network of fecal metabolites found differentially expressed in Africans before and after the dietary switch (‘NA’). Full size image Figure 5: The impact of diet switch on fecal and urinary metabolic reaction networks. ( a – c ) Metabolic reaction networks of metabolites found differentially expressed between different dietary comparisons, created using the MetaboNetworks software [19] using information from the Kyoto Encyclopaedia of Genes and Genomes (KEGG) on the reactions and enzymes within the biological system. The network shows links between metabolites if the reaction entry in KEGG indicates a main reactant pair and the reaction is either mediated by (1) an enzyme linked to human genes, (2) an enzyme linked to genes from identified bacterial groups using the HITChip or (3) it is part of a spontaneous process. The colour of the metabolites indicate whether the metabolite is found in higher concentrations in the urine/feces of individuals consuming an African diet (orange), higher in individuals consuming an African American diet (blue), higher in the African American home environment (light red), higher in the African home environment (green) or whether the metabolites is not significantly associated with any comparison but is part of the metabolic network (white). Two metabolites (alanine and formate) are found with opposite associations in feces and urine ( Table 2 ), these are therefore represented with a grey background colour. A table with full names for each of the abbreviated metabolite names can be found in Supplementary Table 11 . The background shading indicates different interconnected pathways. In the top part of the legend, the colour for each pathway, as represented in the figure, is shown. The bottom part of the legend, with black boxes around text box, indicates the association of each metabolite. ( a ) Global network of changes (‘All’) observed in fecal water and urine, and in any comparison of the different groups. ( b ) Network of fecal metabolites found differentially expressed in African Americans before and after the dietary switch (‘AA’). ( c ) Network of fecal metabolites found differentially expressed in Africans before and after the dietary switch (‘NA’). Full size image Table 2 Fecal and urinary metabolites. Full size table The dietary intervention caused, in tandem with the microbiota changes, substantial modifications in the metabolic phenotypes of both groups ( Table 2 , Fig. 4a ), with Africans demonstrating less metabolic variation and Americans becoming more diverse. This is probably best appreciated from the metabolic pathway analysis ( Fig. 5b,c ) of stool and urine samples from both groups, with colour coding identifying the significant baseline differences, based on integration of the enzymes of bacterial groups identified by HITChip microarray [16] , host metabolic enzymes, and fecal and urinary metabolites by 1 H NMR associated with reactions from the Kyoto Encyclopaedia of Genes and Genomes (KEGG) database. The lower two panels illustrate the significant shifts in metabolic pathways identified in fecal samples after dietary switch, showing mirror image changes reflecting the above, most notably involving reductions in short-chain fatty acids and increases in glycosylated proteins and choline metabolism in Africans, and the unexpected increases in amino acid metabolism in Americans. Consistent with the results of our targeted analyses, the effects on saccharolytic fermentation were reciprocal, with increases in acetate and lactate in Americans and reductions in Africans. Unlike the results obtained from targeted gas chromatography shown of Fig. 2 , the increases in butyrate and propionate measured by global 1 H NMR spectroscopy did not achieve statistical significance, probably possibly due to sample preparation differences between GC and NMR. Again, contrary to expectation, fecal concentrations of colonic branched-chain amino acids, which are likely to be derived from proteolytic fermentation, decreased in Africans given the high-protein western diet for unclear reasons. Global microbe–metabolite associations To investigate this, we performed a partial correlation analysis between genus-level microbes and urine and fecal metabolites ( Fig. 4b ), adjusted for nationality and diet. Although we cannot biologically explain all associations (for example, propionate correlates with enterobacteriaceae and Streptococcus , which are not known to produce propionate), one striking feature was that the metabolite butyrate was exclusively associated with microbial groups that are known to contain butyrate producers, well exemplified by R. intestinalis et rel, E. rectale et rel and C. symbiosum et rel, which are shown in the co-occurrence networks in Fig. 3b , to be enhanced when high-fibre diets were consumed by both population groups. High-fat, low-fibre diets and toxic microbial metabolites It is unlikely that butyrogenesis can alone explain diet-associated cancer risk. Our preceding studies had shown that the higher-fat diet of African Americans was associated with a greater abundance of fecal microbial genes that encode for one of the key enzymes responsible for deconjugation of bile acids (the baiCD gene encodes for the 7α-dehydroxylating enzyme [23] ) as well as their metabolic products, secondary bile acids [5] . Secondary bile acids have been shown to be carcinogenic in experimental models and multiple human studies have shown that their fecal levels are associated with cancer risk [10] , [24] , [25] . Furthermore, there is substantial experimental evidence that the carcinogenic potential of these metabolites is potentiated by colonic butyrate deficiency [26] , [27] , [28] , [29] . Once again, we show that there were reciprocal changes in both baiCD gene abundance and the secondary bile acids, lithocholic and deoxcholic acid, after diet switch, with levels increasing in Africans given the high-fat, western-style diet and reductions in Americans fed the low-fat, traditional African diet ( Fig. 2 , lower panel). Although the use of these functional genes may not cover all the enzymatic pathways of interest, they do provide legitimate tracers for them [30] . Remarkably, Africanization reduced colonic evacuate secondary bile acids by 70% and westernization increased them by 400% ( Supplementary Table 7 ). Dietary fat may influence colon cancer risk through other pathways as illustrated by a recent study in an Il10 −/− mouse model, which showed that a high-fat diet cultivated an increase in the abundance of Biophila wadsworthia , a member of the Desulfovibrionaceae family, which generates hydrogen sulfide via taurine respiration, leading to acute inflammation [31] . Exogenous hydrogen sulfide is a potent genotoxin in vitro [32] . Finally, although no strong evidence has yet been found to indict a specific microbe in colonic carcinogenesis, a recent study found that Fusobacterium nucleatum was enriched in human colon cancer tissue, and suggested that the microbe might promote colorectal neoplasia progression through recruitment of proinflammatory tumour-infiltrating immune cells [33] . Alternatively, members of our group have hypothesized that fusobacteria may promote genotoxity by their ability to convert cysteine to hydrogen sulfide [34] . Figure 2 (upper panel) shows that the presence and activity of both of these microbes may have played a role in the changes in mucosal biomarkers: the high-fibre, low-fat dietary intervention in African Americans was associated with a significant decrease of B. wadsworthia , whereas the low-fibre, high-fat intervention in Africans was associated with an increase of F. nucleatum . We have shown in individuals from high-risk and from low-risk cancer populations that changes in the food content of fibre and fat had remarkable effects on their colonic microbiota and metabonome within 2 weeks, and, critically, that these changes were associated with significant changes in mucosal inflammation and proliferation. Although we cannot claim from our results that these changes in mucosa will result in changes in the development of cancer, there is good experimental evidence that increased epithelial proliferation predicts neoplastic change, because it increases the risk of development of DNA mutations due to the higher rate of exposure of sensitive proliferating cells to luminal carcinogens. The evidence for the use of proliferation biomarkers in humans is based on the known increase in the percentage of epithelial cells engaged in DNA synthesis (measured as ‘proliferation index’) in all premalignant conditions of the gastrointestinal tract, as well as the observed expansion of the proliferative zone, causing a shift of the proliferating cells from the base to the surface of the crypt [35] , [36] , [37] . There is also substantial evidence that chronic inflammation increases cancer risk [38] and it has been observed in human studies that colon cancer is increased fivefold in patients with chronic ulcerative colitis [38] and reduced 50% by anti-inflammatory drugs [39] . In keeping with this, it was noteworthy that our two biomarkers on mucosal inflammation, CD3+ intraepithelial lymphocytes and CD68+ lamina propria macrophages responded in the same direction as our Ki67 proliferative biomarker. CD3 + intraepithelial lymphocytes provide a measure of T-cell activation and, therefore, the pivotal balance between immune activation and quiescence in response to luminal antigens, such as bacteria [40] , [41] , whereas CD68 + lamina propria macrophages play an active role in the persistence of chronic inflammation [42] and neoplastic progression [43] , [44] . Interestingly, the microbial metabolite, butyrate, was shown recently to reduce the responsiveness of lamina propria macrophages to commensal bacteria [45] , suggesting that the dietary change in Americans may have resulted in a decrease in both macrophage numbers and their activity. Our study revealed two unanticipated colonic mucosal findings in rural Africans consuming their usual baseline diets. First, despite the significantly lower epithelial proliferation and population colon cancer rates, mucosal inflammation detected endoscopically, histologically and by immunohistochemistry was more common and pronounced compared with high-risk African Americans ( Fig. 1 ). Second, despite the lower protein intake and lower plasma amino acid levels ( Supplementary Table 9 ), proteolytic fermentation was also increased, releasing metabolites that are known to be inflammatory and pro-carcinogenic [46] . The explanation for these findings is unclear, but may be linked to the high prevalence of chronic parasitic infestations in rural Africans causing inflammation and exudation of mucinous proteins. Of note, schistosoma were incidentally identified in two subjects and a tapeworm segment in another ( Supplementary Fig. 3 ). Intestinal protozoa have been hypothesized to stimulate immunosurveillance against colon cancer [47] . Clearly, further focused investigations of these paradoxical findings are needed, but possible explanations involve the complex associations between inflammation, immunosurveillance and carcinogenesis, and the ability of butyrogenesis to arrest the progression of inflammation to neoplasia. In murine models, lymphocytes can suppress carcinogenesis as part of the process of immunosurveillance, and in patients with tumours, specific intra-tumour lymphocyte markers for Th1 polarization, and cytotoxic and memory T cells have been shown to suppress growth and metastasis, a process termed immunoediting [48] , [49] . Furthermore, T-cell infiltration may suppress or enhance tumorigenesis, depending on the type, density and location of the immune cells. There is substantial experimental evidence, recently reviewed by us [7] , [8] , that the major products of saccharolytic fermentation, acetate, propionate and butyrate have potent anti-neoplastic properties [50] , but butyrate is unique in its maintenance of colonic mucosal health and defense. First, it is the preferred energy source for colonocytes [51] . Second, it has a remarkably wide variety of antineoplastic properties, best exemplified by its function as a histone deacetylase inhibitor [52] , its capacity to downregulate the key canonical W nt -signalling pathway linked to colonic carcinogenesis [53] and its ability to reduce the burden of carcinogens, such as bile acids [28] , [29] , [54] and red meat products [26] . Further studies are needed to explore the intriguing possibility that increased saccharolytic fermentation and butyrogenesis may counter the recognized proliferative properties of T-helper type 17 T cells [55] . Although we have focused on the potential for a high-fibre and high-fat diet to modify metabolic pathways that have been shown experimentally to have an impact on mucosal biomarkers of cancer risk, it must be stressed that a change in one aspect of an otherwise isocaloric diet will inevitably result in a change in another. Consequently, the associated change in animal protein or digestible carbohydrate might also be responsible for the observed mucosal changes. Be that as it may, our results provide fairly substantial evidence for a powerful influence of butyrate on mucosal health and raise hope that an increase in fibre consumption, together with a moderation in fat intake, may reduce the disproportionately high incidence of colon cancer in African Americans and indeed in most westernized communities. Clearly, these suggestions now need to be confirmed by longitudinal studies. With regard to fibre, total quantities may be critical, as fibre supplementation at ≈35 g per day has generally failed to reduce polyp recurrence in clinical trials [56] and recent experimental studies demonstrate that a threshold effect of butyrate availability determines its inhibitory effect on proliferation [52] . Furthermore, human studies by Burkitt [57] concluded that total fibre intake needs to exceed 50 g per day (as in our study) to prevent colon cancer. Our results also raise serious concern that the progressive westernization of African communities may reduce butyrogenesis, allowing their high basal state of chronic inflammation to progress through proliferation to neoplasia [38] , culminating in the emergence of colon cancer as a major health issue [58] . Study design First, the study was submitted to the University of Pittsburgh and University of KwaZulu-Natal Institutional Review Boards for approval. We employed a unique design ( Table 1 and Supplementary Note 1 ), where 20 healthy middle-aged African Americans and 20 rural Africans ( Supplementary Tables 10 : Demographics) from the same communities previously studied [5] were studied first for 2 weeks in their own HE, eating their usual food (HE study), and then again in-house while they were fed the intervention diet for 2 weeks (dietery intervention) study). Consequently, each subject served as his/her own control, which is important given the known wide individual variation in colonic microbiota composition. We chose intervention diets that were at the same time palatable and contained reverse quantities of fibre and fat, such that African Americans would be given ‘African style’ foods increasing their average fibre intake from 14 to 55 g per day and reducing their fat from 35% to 16% of total calories, whereas Africans were given a ‘western-style’ diet reducing their fibre from 66 to 12 g per day and increasing their fat from 16% to 52% ( Supplementary Tables 1–3 ). Cogniscient of the problems of compliance to acute dietary change and the accuracy of dietary recall to estimate actual intakes within the community, we elected to perform all the dietary intervention studies in-house, where meals could be prepared and given under close supervision. With African Americans, participants were housed the University of Pittsburgh Clinical Translational Research Center, and with rural Africans we employed in a rural lodging facility, close to their homes, with full kitchen facilities. Body weights were maintained within 2 kg by adjusting food quantities while keeping the overall macronutrient composition the same. The sampling schedule is given on Table 1 , showing that fresh fecal samples were taken at three intervals during the HE study and again three times after the diet switch. Colonoscopy was performed to identify latent disease, polyps, or cancer, to obtain 3 h colonic evacuates for analysis and biopsies for biomarkers of cancer risk [4] at the beginning of the HE study and end of the dietery intervention study. Full details of the menus, cooking methods and total dietary compositions are given under Supplementary Tables 2, 3 and 4a–c , and Supplementary Note 2 ). Subjects and recruitment Age- and sex-matched healthy volunteers, with the age range 50–65 years, were randomly selected from the African American population in the Pittsburgh region of Pennsylvania and from the rural native South Africans from the rural Kwazulu region. We collaborated with Dr Stephen Thomas, Director of Minority Studies at the University of Pittsburgh School of Public Health, to recruit healthy African American volunteers from the Pittsburgh region, and also advertised the study with the approval of our Institutional Review Board in public areas. In South Africa, volunteers were be recruited through advertisements placed in public community centres, for example, post offices, town halls, civic centres and through the iZulu Community Health Center. Appropriate compensation (as advised by Minority studies and the iZulu Community and ratified by the University of Pittsburgh and KwaZulu-Natal) for time and testing was paid to volunteers for participation. Screening Informed signed consent was taken from each participant. All African volunteers could understand English, but a nurse-translator participated in the consent process to ensure proper understanding of the details of the research procedures. Screening was performed in Pittsburgh at the Clinical Translational Research Center and in Africa at Ngwelezana Hospital outpatient clinic, Empangeni, KwaZulu-Natal, South Africa. A detailed medical history was first taken. With rural Africans, a local bilingual nurse acted as an interpreter. A 20-ml blood sample was taken for full blood count, ESR, electrolytes and urea, albumin, alkaline phosphatase, AST and bilirubin. If the results were normal and if they satisfied the eligibility criteria, they were invited to participate in the study. Subject eligibility Details are given under Supplementary Note 1 . Inclusion criteria were as follows: healthy volunteers, from GI standpoint between 40 and 65 years (age at which colon cancer screening/colonoscopy is recommended in this population) and body mass index between 18 and 35 kg m −2 ( Supplementary Discussion ). Exclusion criteria were as follows: participants pre-colonoscopy were ineligible if they had a history of familial adenomatous polyposis, hereditary non-polyposis colorectal cancer, inflammatory bowel disease or invasive cancer within 5 years before enrollment (h/o adenomatous polyps acceptable). In addition, ineligible participants were individuals with known renal, hepatic or bleeding disorders; previous GI surgery resulting in disturbed gut function due to of loss of bowel or altered anatomy, or any form of chronic GI disease resulting in disturbed gut function, diarrhoea and malabsorption; and individuals with antibiotic use within the past 12 weeks ( Supplementary Discussion ), current steroids use or with diabetes. Exclusion criteria post colonoscopy were detection of previously unrecognized ulceration (with depth and >0.5 cm), stricture, severe inflammation and polyps >1 cm diameter or cancer. Fecal, colonic and mucosal sampling and colonoscopy To synchronize the measurements of the microbiota, the metabolome and the colonic mucosa, the sampling was tied to the preparation for and conduct of a colonoscopy, as previously described [4] , at baseline while on their usual diet (ED1, Table 1 ), and then again at the conclusion of the dietary change (ED2, Table 1 ). In this, fresh fecal samples are collected before colonic evacuation and immediately frozen at −80 °C and the total colonic contents are collected for 3 h during evacuation with a simple polyethylene glycol solution. In this, 2 l of polyethylene glycol (60 g l −1 , average molecular weight 3350g/mol) solution was consumed rapidly as possible over 30 min. We avoided using the commercial preparation ‘Golytely’, as it contains sodium sulfate, which is known to disturb the microbiota composition. Our experience had shown that the quality of bowel preparation with this technique was similar to the more conventional overnight bowel washout. The mucosa health status was assessed by visualization and biopsy. Polyps, when encountered, were removed per standard practice and biopsies were taken from normal mucosa from the proximal (caecum/ascending colon), mid (transverse) and distal (sigmoid) colon at 25 cm from the anal verge. Mucosal samples for immunohistochemistry were collected in formalized saline and for gene expression in RNA later (Qiagen, Germantown, MD) before being stored at −80 °C. Measurement of mucosal biomarkers Histology . Colonic mucosal biopsies were obtained by colonoscopy before and after dietary switch from three different sites (ascending, transverse and descending) and stored in 10% buffered formalin. Later, the biopsy samples were embedded in paraffin and 5-mm sections were cut and stained with either routine haematoxylin and eosin (H&E) or immunohistochemical stains (see below). The histologic findings on the H&E-stained sections were evaluated by one blinded, experienced gastroenterological histopathologist (AK). Measurements focused on the numbers of inflammatory cells and eosinophils in the lamina propria and the numbers of intraepithelial lymphocytes. Scoring of the H&E-stained section was done as shown in Supplementary Table 5a . Any pathologic finding, such as the presence of parasitic organisms, was recorded. Immunohistochemistry Slides for CD3 and Ki67 staining were deparaffinized at 60 °C for 2 h. To inhibit endogenous peroxidase, the slides were pre-treated using 3% hydrogen peroxide/methanol at room temperature (RT) for 10 min, followed by antigen retrieval with 0.2% pepsin solution (P7012, Sigma, 3050 Spruce St, St Louis, MO, USA) at 37 °C for 10 min. Serum Free Protein Block (X0909, Dako, 6392 Via Real, Carpinteria, CA 93013, USA) was used at RT for 10 min. The slides were drained and incubated with primary antibodies CD3 and Ki67 (A0452, 1:100, rabbit polyclonal, Dako; MIB-1, 1:100, mouse monoclonal, Dako), respectively, at RT for 1 h. Secondary detection was applied using Immpress universal antibody Polymer detection kit (MP-7500, Vector Labs, 30 Ingold Road, Burlingame, CA 94010, USA) at RT for 30 min. The slides were stained with DAB substrate kit (SK-4100, Vector Labs) for 10 min and counter stained using Shandon Hematoxylin (6765015, Thermo Scientific, 81 Wyman St, Waltham, MA 02451, USA). Slide staining for CD68 was done on a Ventana Benchmark Ultra slide stainer. Deparaffinized slides were pretreated using the ultra CC1 (950-224, Ventana, 1910 Innovation Park Dr, Tucson, AZ 85755, USA) for 24 min for antigen retrieval. Slides were incubated with the primary antibody CD68 (M087601, 1:100, mouse monoclonal, Clone PG-M1, Dako,) for 32 min RT. The Optivew DAB kit (760-700, Ventana) was used for secondary detection. Quantification of immunohistochemical staining Counting of the proportions of positive staining cells using light microscopy at × 400 magnification was performed by a single investigator (KM), under blinded conditions. To assess inter-observer variability, 40 slides were randomly selected and recounted by a second senior pathologist (AK), showing a concurrence of 88% for Ki67+ and 80% for CD68+ densities. Ki67 The proportion of Ki67-positive staining cells were counted in well-oriented crypts (average/slide 8, range 4–14). Ki67 proliferation rate was defined as the number of Ki67+ cells divided by the total number of crypt cells and were expressed as percentage. The differences were found to be the same in the total crypt and in the upper crypt; hence, only the total crypt proportions are reported here. CD3 Only CD3 + staining intraepithelial lymphocytes were counted in a representative area of at least 300 epithelial cells. The density of intraepithelial lymphocytes was expressed as an index of number of CD3-positive lymphocytes per 100 epithelial cells. CD68 The number of CD68-positive cells (macrophages) within the lamina propria were counted and graded on a scale from 1 to 3: grade 1 (none/rare), grade 2 (scattered superficial collections) and grade 3 (strong, diffuse or band-like infiltrate in the superficial lamina propria) as shown in Fig. 1c . Targeted analysis of fecal and colonic microbes and metabolites of special interest Details of the materials and methods used for the collection, preparation and analysis of fecal samples for targeted analysis of microbes of special interest (real-time quantitative PCR) and their metabolites (Agilent Technologies 6890N Network GC System with a flame-ionization detector for short-chain fatty acids and Shimadzu HPLC–mass spectrometry for quantification using electrospray ionization in negative ion mode by monitoring the (M–H) − ion for bile acids) in African Americans and rural Africans have been previously published [5] . Justification for the use of the BcoA functional gene for butyrate production is that Flint’s group in Aberdeen have demonstrated that although there are a number of different metabolic pathways that use different enzymes that culminate in butyrate synthesis, butyryl-CoA:acetate CoA-transferase, the product of the BcoA gene, is responsible for the last step in butyrate synthesis in the vast majority of intestinal butyrate producers [13] . Similarly, there are other microbial enzymes that participate in bile acid deconjugation, but Wells et al. [23] demonstrated that there was a good correlation between human fecal bacterial dehydroxylating activity measured by fecal dilution assay and their PCR assay for the baiCD gene, which encodes the key enzyme responsible for the bile acid 7α-dehydroxylation pathway. Plasma amino acids Fasting blood concentrations were measured in extracted plasma by reverse-phase C-18 precolumn derivatization HPLC (AccQ·Tag Ultra derivatization, Waters, Milford, MA) as previously described [5] . Statistical analysis Statistical analysis of the group differences in continuous variables was conducted using SPSS 16.0 (SPSS Inc.). The significance of group differences for normally distributed data was assessed with unpaired and paired Student’s t -tests. The non-parametric data were analysed with a Mann–Whitney U -test or Kruskal–Wallis one-way analysis of variance (ANOVA) by ranks for unpaired data and Wilcoxon signed-rank tests for paired data. The significance of the association was evaluated with Spearman’s rank correlation test. A level of P <0.05 was accepted as statistically significant. Data are presented as means ±s.e. Complex microbiota and metabonome data were analysed by several multivariate ordinations detailed below (principal component analyses and non-metric multidimensional scaling), Kruskal–Wallis independent tests and multivariate ANOVA with Bonferroni correction. Global analysis of the microbiota composition and diversity We chose the HITChip phylogenetic microarray for the global profiling of microbiota composition. It has been demonstrated that the HITChip analysis of fecal samples provides highly concordant results concerning the microbiota composition when compared with 16S rRNA gene or metagenome sequencing [59] , [60] , [61] , [62] , as it allows deep profiling of phylotypes at high resolution, down to <0.1% relative abundance, corresponding to a duplicated set of 100,000 pyrosequencing reads per sample with very high reproducibility (>98%) [59] and at considerably lower cost. HITChip analysis DNA was isolated from fecal or colonic samples and subsequently used for phylogenetic profiling of the intestinal microbiota using the HITChip phylogenetic microarray [16] . Standardized quality control was maintained through our library of a duplicated set of 3,631 probes targeting the 16S rRNA gene sequences of over 1,000 intestinal bacterial phylotypes. Briefly, the full-length 16S rRNA genes were amplified, and PCR products were transcribed in vitro into RNA, labelled with Cy3 and Cy5, and fragmented. Hybridizations were performed in duplicate and data were extracted from microarray-scanned images using Agilent Feature Extraction software, version 10.7.3.1 ( http://www.agilent.com ). Array normalization was performed as previously described, using a set of custom R scripts ( http://r-project.org ) and stored in a custom MySQL database ( http://www.mysql.com ). Duplicate hybridizations with a Pearson correlation >98% were considered for further analysis. Microbiota profiles were generated by pre-processing the probe-level measurements with minimum–maximum normalization and the frozen Robust Probabilistic Averaging probe summarization [62] , [63] into three phylogenetic levels: level 1, defined as order-like 16S rRNA gene sequence groups; level 2, defined as genus-like 16S rRNA gene sequence groups (sequence similarity >90%); and level 3, phylotype-like 16S rRNA gene sequence groups (sequence similarity >98%). In the present work, we primarily focus on the genus-level (level 2) variation. Significance of the differences between the time points ( Fig. 3a ) were estimated based on a (paired) linear model for microarrays (limma) with the threshold of false discovery rate (FDR)<0.2 estimated based on Benjamini–Hochberg procedure and a minimum fold change of 25% (0.1 at the Log10 scale) [64] . Microbial co-occurrence network analysis We constructed the co-occurrence networks between the 130 genus-like bacterial groups based on their logarithmic abundances (HITChip log10 signal) within each treatment group (African Americans and Native Africans; before and after the dietary intervention). For a robust correlation analysis, we applied the SparCC algorithm using 20 iterations and with 50 bootstrap data sets for significance testing, followed by q -value [65] correction of the pseudo P -values from the bootstrap analysis. We focused on the significant (| r |>0.5; q <0.01) correlations between the genus-like groups where a qualitative change (change of sign) in the correlation was observed following the dietary intervention. To ensure robust analysis, we included only the correlations that changed drastically in the intervention, with a difference of >1 between the correlation values before and after intervention (so that the correlations would change for instance from −0.5 to 0.5, or higher). This provided a list of genus-like bacteria that had significant changes in their mutual correlation networks following the dietary intervention in either rural African or African American group. To simplify interpretation, we clustered the associated genus-like groups into coherent network modules with complete-linkage hierarchical clustering based on the SparCC correlations. We defined a module as a connected sub-network where the correlations between all genus-like groups within the module are r >0.5. Networks were visualized using the network visualization and exploration platform Gephi [66] . The resulting modules are highlighted in Fig. 3b . Global analysis of the metabolome: sample preparation for NMR spectroscopic analysis All urinary samples were thawed at RT and vortexed for 10 s. A total of 400 μl of urinary sample was thoroughly mixed with 250 μl of 0.2 M sodium phosphate buffer containing 20% D 2 O, pH 7.4, 0.01% 3-(trimethylsilyl)-[2,2,3,3-2H 4 ]propionic acid sodium salt and 3 mM sodium azide (NaN 3 ). The mixture was subsequently centrifuged at 10,000 g for 10 min and 600 μl of supernatant was transferred into an NMR tube with an outer diameter of 5 mm. Approximately 200 mg of wet fecal sample was mixed with 600 μl of H 2 O (HPLC grade) in a 1.5-ml Eppendorf tube. A cycle of 30-s vortexing, 5-min sonicating at 4 °C and 30-s vortexing was then carried out on the mixture, followed by centrifuging at 10,000 g for 10 min. A total of 400 μl of supernatant was added into a 1.5-ml Eppendorf tube containing 250 μl of aforementioned sodium phosphate buffer, vortexed and spun at 10,000 g for 10 min. An amount of 600 μl of supernatant was put into an NMR tube. 1 H NMR spectroscopy 1 H NMR spectra of urinary and fecal water extract samples were acquired using a Bruker 600 MHz spectrometer (Bruker, Rheinstetten, Germany) at the operating 1 H frequency of 600.13 MHz at a temperature of 300 K. An NMR pulse sequence (recycle delay -90°- t 1 -90°- t m -90°-acquisition) and standard parameters were used to obtain standard one-dimensional 1 H NMR spectral data as described in Beckonert et al. [67] Multivariate statistical data analysis 1 H NMR spectra of urine and fecal extracts were automatically phased, referenced to 3-(trimethylsilyl)-[2,2,3,3- 2 H 4 ]propionic acid sodium salt at 1 H δ 0.00 and baseline-corrected using an in-house developed MATLAB script (Dr Tim Ebbels, Imperial College London). The processed NMR spectra ( 1 H δ 0 to 10) were imported to MATLAB (R2012a, MathWorks) and digitized into 20k data points with a resolution of 0.0005 p.p.m. using an in-house developed script. The water peak region in urine (4.7–5.14 p.p.m.) and fecal water spectra (4.7–5.18 p.p.m.) were removed to minimize the effect of the disordered baseline caused by water suppression. In addition, regions ( 1 H 0–0.3) in urine spectra and regions ( 1 H 0–0.25) in fecal water spectra containing only noise were therefore removed, together with the urea signal in urine ( 1 H 5.48–6.24). Because of the heavy peak shifting in urinary spectra, a recursive segment-wise peak alignment method was applied, to improve metabolic biomarker recovery [68] . Probabilistic quotient normalization was subsequently performed on the resulting data sets, to account for dilution of complex biological mixtures [69] . Principal component analysis and orthogonal partial least-squares discriminant analysis was carried out with a unit variance scaling method in SIMCA (P+13.0) and MATLAB software. P -values of metabolites were calculated using ANOVA and FDR was also calculated for each metabolite marker [70] . For the two-way clustered heatmap ( Fig. 4b ) between fecal microbiota and metabolite concentrations in urine and feces, the partial correlation was calculated for each phylotype and metabolite. The correlation was adjusted for country and dietary intervention to account for baseline differences. A pFDR cutoff value of 0.3 was used to define the significance (denoted by ‘+’), to account for the different numbers of samples in each data set. For each data set (microbiota, fecal metabolites and urinary metabolites), the data were clustered using hierarchical cluster analyses with complete linkage. The optimal number of clusters was chosen as the splitting that maximized the modularity using the correlation as weight of each edge in the network. Metabolic reaction network generation Using the freely available MetaboNetworks software [19] reactions that occur spontaneously or by means of enzymes linked to human and/or bacterial genomes were identified in the KEGG. All complete genome sequences listed in KEGG that could be associated to the bacterial groups represented on the HITChip were included in creating the database, resulting in a total of 817 bacterial genomes included in the database. Next, the software was used to construct a shortest-path metabolic reaction network between all (fecal and urinary) metabolites significantly different in any of the different dietary comparisons. From this ‘global network’, two sub-graphs were generated for each of the two dietary switches using significantly associated fecal metabolites. To highlight the differential expression of the metabolites associated with specific pathways, the background shading was added to the graphs to indicate the different interconnecting pathways ( Fig. 5a–c ). The abbreviations and full names of these metabolites can be found in Supplementary Table 11 . Accession codes: Microbiome and metabolome data have been deposited in the Dryad Digital Repository: http://dx.doi.org/10.5061/dryad.1mn1n. How to cite this article: O’Keefe, S. J. D. et al. Fat, fiber and cancer risk in African Americans and rural Africans. Nat. Commun. 6:6342 doi: 10.1038/ncomms7342 (2015).